Ca2+-dependent phospholipid scrambling by a reconstituted TMEM16 ion channel Phospholipid (PL) scramblases disrupt the lipid asymmetry of the plasma membrane, externalizing phosphatidylserine to trigger blood coagulation and mark apoptotic cells. Recently, members of the TMEM16 family of Ca 2+ -gated channels have been shown to be involved in Ca 2+ -dependent scrambling. It is however controversial whether they are scramblases or channels regulating scrambling. Here we show that purified afTMEM16, from Aspergillus fumigatus , is a dual-function protein: it is a Ca 2+ -gated channel, with characteristics of other TMEM16 homologues, and a Ca 2+ -dependent scramblase, with the expected properties of mammalian PL scramblases. Remarkably, we find that a single Ca 2+ site regulates separate transmembrane pathways for ions and lipids. Two other purified TMEM16-channel homologues do not mediate scrambling, suggesting that the family diverged into channels and channel/scramblases. We propose that the spatial separation of the ion and lipid pathways underlies the evolutionary divergence of the TMEM16 family, and that other homologues, such as TMEM16F, might also be dual-function channel/scramblases. Phosphatidylserine (PS) is normally sequestered in the inner leaflet of the plasma membrane [1] . The surface exposure of PS marks apoptotic cells for phagocytic clearance and triggers blood clotting in activated platelets [2] , [3] . PS exposure is mediated in part by Ca 2+ -dependent lipid scramblases that flip lipids bidirectionally across the plasma membrane [3] . Despite their importance in cell physiology, the molecular identity of the scramblases has eluded researchers for decades [3] . Recently, TMEM16F, a member of the TMEM16 family of Ca 2+ -gated ion channels [4] , [5] , [6] , was shown to be important for Ca 2+ -dependent exposure of PS [7] , [8] , [9] , [10] . Mutations in TMEM16F cause Scott syndrome, a bleeding disorder associated with defective lipid scrambling in platelets [7] , [11] , [12] . Deletion of TMEM16F in mice leads to prolonged bleeding and impaired PS scrambling [8] , as well as decreased bone mineralization [9] . It is controversial, however, whether TMEM16F and other TMEM16 family homologues are scramblases rather than channels [7] , [13] , or whether TMEM16F is a cation channel regulating a yet unidentified scramblase [8] , or one of several types of anion channels with diverse functional properties, such as activation by volume [14] , depolarizing voltages [15] or Ca 2+ (refs 16 , 17 , 18 , 19 ). TMEM16F was proposed to form a Ca 2+ -gated cation channel in megakaryocytes and in heterologous systems, but its overexpression in several cell lines failed to induce Ca 2+ -dependent PS scrambling, suggesting that TMEM16F itself was not a scramblase [8] . In contrast, other groups reported that heterologous expression of TMEM16F, and of some other TMEM16 family members, could induce Ca 2+ -dependent phospholipid (PL) scrambling [7] , [13] , [17] . Thus, although several independent lines of evidence indicate that some TMEM16 homologues are implicated in Ca 2+ -dependent lipid scrambling, there is disagreement on whether they are scramblases or channels that regulate scrambling [7] , [8] , [9] , [10] , [12] , [13] , [17] . A biochemically pure preparation and a direct assay for scrambling are needed to offer definitive proof of activity in the form of the functional reconstitution of a purified protein. Our initial attempts to purify and reconstitute TMEM16F showed that the protein was unstable. We then screened the genomes of eukaryotic organisms for homologues that could be purified and functionally reconstituted. We were successful with three other TMEM16 homologues: hTMEM16A, the founding member of the TMEM16 family that forms Ca 2+ -activated Cl − channels in vivo [4] , [5] , [6] and in vitro [20] ; Ist2p, the TMEM16 homologue involved in intracellular membrane contacts in the yeast Saccharomyces cerevisiae [21] , [22] ; and afTMEM16, a previously uncharacterized homologue from Aspergillus fumigatus . Although the overall sequence homology among TMEM16 family homologues is low, the conservation in four putative transmembrane domains, TM1, 2, 5 and 7a/b, is much higher ( Supplementary Fig. S1 and Supplementary Table S1 ). Interestingly, in these regions the degree of homology of afTMEM16 to the mammalian TMEM16 is much higher than to Ist2p ( Supplementary Fig. S1 and Supplementary Table S1 ), suggesting that it’s function(s) as a TMEM16 family member might be better conserved. We reconstituted the purified proteins and tested whether they directly mediate lipid scrambling. Remarkably, we found that afTMEM16 is a dual-function protein: it is a Ca 2+ -gated ion channel and a Ca 2+ -dependent PL scramblase. Our data provide the first direct demonstration that the TMEM16 family encodes the long-sought Ca 2+ -dependent scramblases. Purified afTMEM16 forms Ca 2+ -gated ion channels We purified afTMEM16 to homogeneity ( Supplementary Fig. S2a ) and reconstituted it into vesicles. After fusing these vesicles to preformed planar lipid bilayers, we observed single channels of high conductance, ~300 pS ( Fig. 1a–c ) ( n= 7). The channels were poorly selective; their currents reversed at ~−9 mV in the presence of a tenfold KCl gradient ( Fig. 1c ), indicating a minor cationic preference of P K / P Cl ~1.5. The channels were gated by both voltage and Ca 2+ : the open probability increased at depolarizing potentials, reaching ~1 at V> −50 mV ( Supplementary Fig. S3 ) and removing Ca 2+ from the cis -chamber reduced channel activity at −100 mV ( Fig. 1b ). No channels were detected in 35 recordings, wherein liposomes reconstituted with mock preparations were fused to the bilayers ( Supplementary Table S2 ). 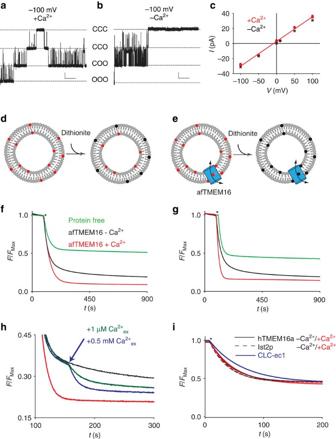Figure 1: Ion transport and lipid scrambling by afTMEM16. (a,b) Recording of three afTMEM16 channels at −100 mV with 0.5 mM Ca2+(a) or 1 mM EDTA on thecis-side (b). Open (O) and closed (C) states are indicated by dashed lines. Channels with similar properties were seen inn=7 independent bilayers. Perfusion to 1 mM EDTA could be performed only in two out of seven bilayers, and resulted in a similar reduction in activity. Scale bar (horizontal), 10 s; scale bar (vertical), 10 pA. (c) Current–voltage plot of afTMEM16 in the presence of a tenfold KCl gradient with (red squares) or without (black crosses) Ca2+. Red line: linear fit withVrev=−8.3±2.7 mV. The points represent the average of two to seven independent recordings. Error bars, s.e.m. (d,e) Dithionite-based scramblase assay. NBD lipids (red) are irreversibly reduced (black) by dithionite. In protein-free liposomes only outer-leaflet fluorophores are reduced (d), whereas in afTMEM16 proteoliposomes all fluorophores are inactivated (e). (f,g) Representative traces of the fluorescence loss of NDB-PS (f) or NBD-PE (g) after addition of dithionite: green, protein-free liposomes with 0.5 mM Ca2+; afTMEM16 proteoliposomes with 0.5 mM Ca2+(red) or in 0 mM Ca2+(black). (h) Scrambling in symmetrical 0.5 mM Ca2+(red) or 0 mM Ca2+(black). The blue and green traces correspond to experiments started in symmetrical 0 mM Ca2+, and att~160 s, 0.5 mM (blue) or 1 μM (green) Ca2+exis added to the extraliposomal solution. Dithionite was added att=100 s in all cases and is not shown. For clarity, only theF/Fmaxinterval between 0.15 and 0.45 is shown. (i) Fluorescence loss in liposomes reconstituted with CLC-ec1 (blue), hTMEM16A (solid lines) or Ist2p (dashed lines) in the presence (red) or absence (black) of Ca2+. *Addition of dithionite. Figure 1: Ion transport and lipid scrambling by afTMEM16. ( a , b ) Recording of three afTMEM16 channels at −100 mV with 0.5 mM Ca 2+ ( a ) or 1 mM EDTA on the cis -side ( b ). Open (O) and closed (C) states are indicated by dashed lines. Channels with similar properties were seen in n= 7 independent bilayers. Perfusion to 1 mM EDTA could be performed only in two out of seven bilayers, and resulted in a similar reduction in activity. Scale bar (horizontal), 10 s; scale bar (vertical), 10 pA. ( c ) Current–voltage plot of afTMEM16 in the presence of a tenfold KCl gradient with (red squares) or without (black crosses) Ca 2+ . Red line: linear fit with V rev =−8.3±2.7 mV. The points represent the average of two to seven independent recordings. Error bars, s.e.m. ( d , e ) Dithionite-based scramblase assay. NBD lipids (red) are irreversibly reduced (black) by dithionite. In protein-free liposomes only outer-leaflet fluorophores are reduced ( d ), whereas in afTMEM16 proteoliposomes all fluorophores are inactivated ( e ). ( f , g ) Representative traces of the fluorescence loss of NDB-PS ( f ) or NBD-PE ( g ) after addition of dithionite: green, protein-free liposomes with 0.5 mM Ca 2+ ; afTMEM16 proteoliposomes with 0.5 mM Ca 2+ (red) or in 0 mM Ca 2+ (black). ( h ) Scrambling in symmetrical 0.5 mM Ca 2+ (red) or 0 mM Ca 2+ (black). The blue and green traces correspond to experiments started in symmetrical 0 mM Ca 2+ , and at t ~160 s, 0.5 mM (blue) or 1 μM (green) Ca 2+ ex is added to the extraliposomal solution. Dithionite was added at t =100 s in all cases and is not shown. For clarity, only the F / F max interval between 0.15 and 0.45 is shown. ( i ) Fluorescence loss in liposomes reconstituted with CLC-ec1 (blue), hTMEM16A (solid lines) or Ist2p (dashed lines) in the presence (red) or absence (black) of Ca 2+ . *Addition of dithionite. Full size image afTMEM16 is a Ca 2+ -dependent PL scramblase To assay scrambling, we reconstituted afTMEM16 into liposomes containing trace amounts of PLs bearing a nitrobenzoxadiazole (NBD) fluorophore and measured the time course of fluorescence loss due to the addition of the membrane-impermeant anion dithionite [23] , [24] . In liposomes with no scramblases, the fluorescence decay reaches 50%, as only outer-leaflet NBD-PLs (NBD-PLs) are reduced ( Fig. 1d,f , green trace), and is well described by a single exponential function with τ 0 ~ 20 s ( n≥ 6 for each lipid) regardless of the presence of Ca 2+ in solution and of the specific lipid used. In scramblase-equipped liposomes, the extent of fluorescence loss is expected to reach 100%, as NBD lipids flip from the inner to the outer leaflet ( Fig. 1e ). We tested whether afTMEM16 scrambles NBD-labelled PS (NBD-PS) and phosphatidylethanolamine (NBD-PE). In proteoliposomes reconstituted with high copy numbers of afTMEM16 in the presence of saturating Ca 2+ , we observed ~85% fluorescence reduction ( Fig. 1f , red trace). This suggests that afTMEM16 is a scramblase. Remarkably, Ca 2+ modulated the rate of lipid scrambling. In high Ca 2+ , the fluorescence decay reached a plateau in ~100 s after the addition of dithionite ( Fig. 1f,g red trace), with slightly different kinetics for the different substrates τ (Ca 2+ , PS)=37±2 s ( n= 3) and τ (Ca 2+ , PE)=19±1 s ( n= 10). Removal of Ca 2+ slowed the process so that steady state was not reached after 900 s ( Fig. 1f,g , black trace). This is reflected in the appearance of a second kinetic component in the fluorescence decay time course, with τ Slow (0 mM Ca 2+ , PS)>300 s ( n= 3) and τ Slow (0 mM Ca 2+ , PE)>400 s ( n= 12). The two components in the fluorescence decay do not reflect two distinct processes mediated by afTMEM16, rather they are a complex function of the rates of scrambling and dithionite reduction. At low Ca 2+ , the two components are sufficiently different that we can assign the fast one to the dithionite reduction of the outer leaflet and the slow one to the progressive exposure of inner-leaflet lipids to the outside. In contrast, at high Ca 2+ the fluorescence decay is well described by a single exponential function with a time constant, similar to that seen in protein-free liposomes. Therefore, at high Ca 2+ the fluorescence decay is rate limited by the chemical reduction of the NBD fluorophore by dithionite rather than by lipid scrambling. If we assume that an average liposome contains ~10 6 lipids [25] and ~5 copies of purified afTMEM16 (see below), then we can estimate that the rate of lipid flipping in 0 mM Ca 2+ is ~400 lipid per second and that in saturating Ca 2+ it is >10 4 lipid per second, a >20-fold increase in rate. The Ca 2+ dependence of the rate of lipid scrambling is readily visualized by measuring the fluorescence decay in liposomes prepared in symmetrical 0 mM Ca 2+ and to which, ~60 s after the addition dithionite, 0.5 mM Ca 2+ was added to the extraliposomal solution ( Fig. 1h ). The sudden increase in Ca 2+ ex ‘turns on’ the scramblases with an extracellular ligand-binding site and the rate of fluorescence decay increases ~20-fold ( Fig. 1h ). A comparable increase in rate was visible upon adding 1 μM Ca 2+ ex ( Fig. 1h ), suggesting that afTMEM16 has a micromolar Ca 2+ sensitivity. These results suggest that afTMEM16 is a PL scramblase and that Ca 2+ modulates its flipping rate by more than 20-fold. It is important to note that the incomplete loss of fluorescence suggests that a small fraction of vesicles is refractory to protein insertion, as previously reported [24] , [26] , [27] . We found that among all tested reconstitution conditions, the value of the refractory pool varies ~2-fold, from a minimum value of ~13%, for vesicles containing NBD-phosphatidylcoline (NBD-PC), to a maximum value of ~30%, for vesicles prepared in 300 mM N-methyl- D -glucamine-Cl (NMDG-Cl). However, for any one condition the variability is limited; for example, in 0 mM Ca 2+ it varies from 18 to 23% ( n= 12) and in 0.5 mM Ca 2+ it varies between 14 and 18% ( n= 10). This is consistent with the notion that liposome size and properties are affected by the composition of the buffer and of the lipid membrane [28] , [29] . To rule out the possibility that the fluorescence decay reflects dithionite permeation through afTMEM16 rather than lipid scrambling, we prepared liposomes in the presence of 60 μM NBD-glucose, removed the external NBD-glucose via a spin column and monitored the time course of fluorescence decay after dithionite addition. If dithionite permeates through afTMEM16, it will gain access to the NBD-glucose trapped inside the vesicles and reduce the fluorophore. In this case, we expect to see a >80% drop in fluorescence ( Supplementary Fig. S4a ), with kinetics similar to those seen for scrambling in the presence of 0.5 mM Ca 2+ ( Fig. 1g,h ). In contrast, if dithionite does not permeate through afTMEM16 then the total fluorescence should remain nearly constant ( Supplementary Fig. S4b ). This is the case: in afTMEM16 proteoliposomes, the fluorescence decays very slowly and at a rate that is nearly indistinguishable from that seen in protein-free liposomes ( Supplementary Fig. S4c ), ~0.02% of total fluorescence per second in both cases. The initial jump immediately following the addition of dithionite reflects the incomplete removal of NBD-glucose from the extraliposomal solution by the spin column. Finally, to rule out the possibility that scrambling mediated by afTMEM16 is a process specific to the modified reporter lipids, in which one fatty acid chain has been replaced with a short chain bearing an NBD fluorophore, we examined the dependence of the rate of fluorescence decay on the concentration of NBD-PE. If afTMEM16 specifically transports only NBD-labelled lipids, then the time constant of fluorescence decay should depend strongly on the concentration of NBD-PE. If, on the other hand, all the lipids in a liposome are scrambled by afTMEM16, then the kinetics should be independent from the NBD-PE concentration. These measurements were performed in 0 mM Ca 2+ , a regime where the rate of lipid scrambling is ~20-fold slower than the rate of dithionite reduction of the NBD fluorophore ( Fig. 1f–h ), so that the two processes can be readily separated. We found that upon changing the NBD-PE concentration 100-fold (from 0.05 to 5% of total lipid), the time constants of fast and slow decay are nearly unaffected ( Supplementary Fig. S5a,b ), τ Slow is ~380 s at 0.05% to ~320 s at 5%, indicating that scrambling is not specific for NBD-labelled lipids. Thus, we conclude that afTMEM16 scrambles all the lipids contained in each vesicle. To further strengthen our conclusion that afTMEM16 is a PL scramblase, we used fatty-acid-free BSA as a topological probe of scrambling ( Supplementary Fig. S6a ). BSA extracts NBD-PLs and quenches their fluorescence by ~50% [24] , [30] . Consistent with expectations, we saw ~27% fluorescence reduction upon BSA addition to protein-free liposomes and ~53% reduction in afTMEM16 proteoliposomes with Ca 2+ -dependent kinetics ( Supplementary Fig. S6b ). Therefore, the dithionite- and BSA-based assays independently demonstrate that afTMEM16 is a Ca 2+ -dependent PL scramblase. Not all TMEM16 homologues mediate lipid scrambling We next tested whether lipid scrambling is a general property of all TMEM16 family members or whether the presence of an integral membrane protein might disturb the lipid bilayer enough to induce scrambling. First, we verified that we do not detect lipid movement in proteoliposomes containing CLC-ec1, a CLC-type H + /Cl − exchanger with no physiological connection to PL scrambling ( Fig. 1i ). This is consistent with numerous previous reports showing that the mere presence of a membrane protein in vesicles does not promote rapid transbilayer movement of lipids [24] , [31] , [32] . Then, we purified and reconstituted hTMEM16A ( Supplementary Fig. S2b ) and Ist2p ( Supplementary Fig. S2c ), and found that neither protein mediates lipid scrambling regardless of the presence of Ca 2+ ( Fig. 1i ). Thus, our data suggests that not all TMEM16 homologues are PL scramblases. afTMEM16 is a dual-function channel/scramblase To eliminate the possibility that either the channel or the scramblase activity is mediated by a co-purified contaminant rather than by afTMEM16, we examined the dependencies of these activities on the total protein reconstituted. If a channel and a scramblase are co-purified and are present in different numbers, then the fractions of liposomes containing 0 copies of a protein, f 0 , for the two activities should follow a Poisson distribution [24] , [26] and diverge at low protein densities ( Supplementary Fig. S7a ). In contrast, if afTMEM16 is a dual-function protein, then the two fractions should co-vary. We exploited the poor ion selectivity of afTMEM16 to develop a ‘flux’ assay for its ion channel activity. Liposomes containing one or more open afTMEM16 channels should not maintain a KCl gradient, whereas protein-free liposomes (or those with closed channels) should ( Fig. 2a ). Therefore, the Cl − content of liposomes exposed to a large KCl gradient is a direct measure of the channel activity of afTMEM16 ( Fig. 2b ). In the presence of Ca 2+ , afTMEM16 proteoliposomes retain only ~20% ( n= 17) of the Cl − content of protein-free liposomes ( Fig. 2b,c ). The non-zero residual Cl − content is consistent with the fraction of reconstitution-refractory liposomes seen in scrambling assays ( Fig. 1f,g ). In contrast, the Cl − content of proteoliposomes in 0 mM Ca 2+ was ~75% ( n= 16; Fig. 2b,c ), consistent with the channels being mostly closed. These bulk measurements recapitulate the properties of single afTMEM16 channels seen in bilayers ( Fig. 1 and Supplementary Fig. S3 ). We determined f 0 at different protein concentrations using flux and scrambling assays, and found that they co-vary ( Fig. 2d ), with p 0 values of ~0.4 μg protein per mg lipid, indicating that both ion channel and lipid scramblase activities are mediated by afTMEM16. 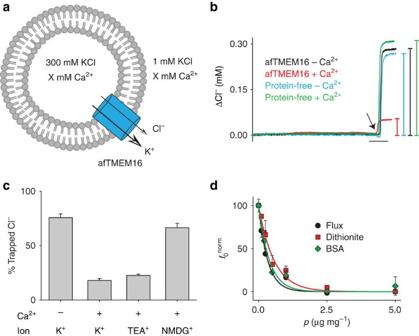Figure 2: afTMEM16 is a dual-function protein. (a) Cl−efflux assay. (b) Measure of Cl−content in protein-free liposomes in 0.5 (green) or 0 (blue) mM Ca2+and in afTMEM16 proteoliposomes with 0.5 (red) or 0 (black) mM Ca2+. Arrow denotes the addition of detergent to solubilize liposomes. Vertical bars represent the value of ΔCl−. Scale bar, 15 s. (c) Fraction of trapped Cl−in proteoliposomes reconstituted with or without 0.5 mM Ca2+and with K+, TEA+or NMDG+. (d) Protein dependence off0normmeasured by flux (black) and lipid scrambling (dithionite (red) or BSA (green) assays. Solid lines are fits to equation (4) withp0(Flux)=0.35±0.06,p0(Dithionite)=0.51±0.07andp0(BSA)=0.40±0.06 μg protein per mg lipid. Each data point represents the average of three to six independent experiments and the error bars are s.e.m. The errors on the fit parameters are the uncertainties of the fits. Figure 2: afTMEM16 is a dual-function protein. ( a ) Cl − efflux assay. ( b ) Measure of Cl − content in protein-free liposomes in 0.5 (green) or 0 (blue) mM Ca 2+ and in afTMEM16 proteoliposomes with 0.5 (red) or 0 (black) mM Ca 2+ . Arrow denotes the addition of detergent to solubilize liposomes. Vertical bars represent the value of ΔCl − . Scale bar, 15 s. ( c ) Fraction of trapped Cl − in proteoliposomes reconstituted with or without 0.5 mM Ca 2+ and with K + , TEA + or NMDG + . ( d ) Protein dependence of f 0 norm measured by flux (black) and lipid scrambling (dithionite (red) or BSA (green) assays. Solid lines are fits to equation (4) with p 0 (Flux)=0.35±0.06, p 0 (Dithionite)=0.51±0.07and p 0 (BSA)=0.40±0.06 μg protein per mg lipid. Each data point represents the average of three to six independent experiments and the error bars are s.e.m. The errors on the fit parameters are the uncertainties of the fits. Full size image Comparison of afTMEM16 with mammalian TMEM16 channels In addition to sensitivity to Ca 2+ and voltage ( Fig. 1 and Supplementary Fig. S3 ), afTMEM16 channels share a number of properties with TMEM16A and TMEM16F [4] , [5] , [6] , [8] , [33] , [34] , [35] . Our Poisson-dilution measurements ( Fig. 2d ) [26] suggest that the functional afTMEM16 unit has a molecular mass of ~190 kDa, indicating that, similar to TMEM16A [36] , [37] , afTMEM16 forms dimers in membranes ( Supplementary Fig. S7b ). We found that afTMEM16 is a nearly non-selective ion channel ( Figs 1 ), with P K / P Cl ~1.5. Although this poor selectivity is unusual for better characterized channels [38] , most TMEM16 ion channels appear to be poorly selective. For example, the anion/cation selectivity of TMEM16A is only ~0.15 (refs 5 , 8 , 35 ) and at least one of its splice variants has an even greater permeability to cations [34] . Similarly, cationic currents associated with TMEM16F also appear to be poorly selective, P K / P Cl ~7, and a point mutation decreases their selectivity to ~2.2 (ref. 8 ), a value close to that of afTMEM16. Finally, the anionic currents associated with TMEM16F also display significant cation permeabilities, P Na / P Cl ~0.3 (ref. 19 ). The afTMEM16 pore appears to be large; our permeability experiments show that TEA + permeates through the channel, whereas NMDG + appears to be excluded ( Fig. 2c ), suggesting that the radius of the narrowest portion of the afTMEM16 pore is between 4 and 6.5 Å. Similarly, TMEM16A and 16F also allow the permeation of large ions, such as gluconate − (ref. 34 ) and NMDG + (ref. 8 ), respectively, indicating that these other family homologues also have pores of wide diameters. Despite these similarities, we note that the single-channel conductance of afTMEM16 is much higher than that of TMEM16A or 16F [6] , [8] , and the channel remains open at negative voltages ( Fig. 1a,b and Supplementary Fig. S3 ). The physiological implications of the high conductance and poor selectivity of afTMEM16 are unclear, as we do not know its role in the physiology of its native organism, the pathogenic fungus A. fumigatus . Further work will be required to elucidate this point. Similarity of afTMEM16 to mammalian scramblases We found that afTMEM16 recapitulates the known properties of mammalian Ca 2+ -dependent scramblases: Ca 2+ -dependent, rapid and poorly selective lipid movement between membrane leaflets [39] . Removal of Ca 2+ slows afTMEM16-mediated scrambling by >20-fold ( Fig. 1f,g ), from >10 4 to ~400 lipid per second. We also found that afTMEM16 mediates the Ca 2+ -dependent transport of a variety of lipids, albeit at different rates: NBD-PS ( Fig. 1f ), NBD-PE ( Fig. 1g ) and NBD-PC ( Supplementary Fig. S8a ), as well as PE bearing the NBD fluorophore on the headgroup, N -NBD-DPPE ( Supplementary Fig. S8b ), NBD-glucosylceramide ( Supplementary Fig. S8c ) and the cationic lipid DOTAP ( Supplementary Fig. S8d ). As we cannot determine the absolute rate of lipid scrambling in the presence of Ca 2+ , we quantified the lipid selectivity of afTMEM16 by measuring the fluorescence at a fixed time point chosen to be equal to three times the τ 0 of fluorescence decay measured in protein-free liposomes, F *. At this time point, the reduction of the outer-leaflet lipids by dithionite is ~95% complete so that F *-values below 0.5 indicate PL scrambling ( Supplementary Fig. S9a ). For example, F *(PC, 0 mM Ca 2+ )=0.38±0.02, indicating that after 60 s from the addition of dithionite and in the absence of Ca 2+ ~20% of the inner leaflet, NBD-PC lipids have been reduced ( Supplementary Fig. S9b ). In the same time interval in the presence of Ca 2+ , F *(PC, Ca 2+ )=0.09±0.01, indicating that ~80% of the inner-leaflet lipids have been scrambled. Our results suggest that afTMEM16 displays a moderate selectivity of PC>PE>PS~glucosylceramide>DOTAP ( Supplementary Fig. S9b ). Our results demonstrate that afTMEM16 is a novel dual-function protein with the characteristics of Ca 2+ -gated TMEM16 ion channels and Ca 2+ -dependent PL scramblases. As afTMEM16 has the same number of transmembrane segments as the channel-only homologue TMEM16A ( Supplementary Fig. S1 ), we can exclude that during evolution a TMEM16 channel became fused to a ‘scramblase’ domain. Therefore, both activities coexist within the TMEM16 transmembrane scaffold, suggesting that they might be coupled. To test this hypothesis, we asked whether the same Ca 2+ -binding site controls both transport functions and whether the ion and lipid pathways coincide. A common Ca 2+ -binding site regulates ion and lipid transport We first characterized the Ca 2+ dependence of afTMEM16’s channel and scramblase activities. The rate of afTMEM16-mediated lipid scrambling increased with Ca 2+ ( Fig. 3a ), with a mid-point of activation of ~0.4 μM ( Fig. 3b ). Similarly, 0.5 μM Ca 2+ was sufficient to open the afTMEM16 channel in flux assays ( Fig. 3c ). The two activities share a similar selectivity for divalent cations: Ca 2+ fully activates both transport functions, Mn 2+ , Sr 2+ and Ba 2+ elicit intermediate responses, whereas Mg 2+ and Cd 2+ fail to activate either ( Fig. 3d–f ). Thus, both transport functions of afTMEM16 share the same apparent divalent selectivity of: Ca 2+ >Mn 2+ ~Sr 2+ >Ba 2+ >Cd 2+ ~Mg 2+ ( Fig. 3d–f ). 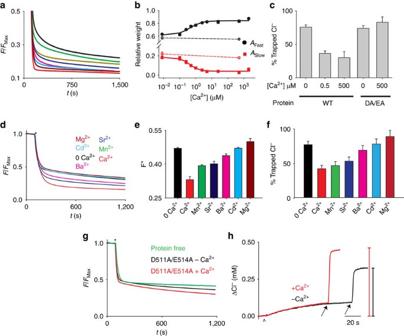Figure 3: A shared Ca2+ binding site regulates channel gating and phospholipid scrambling by afTMEM16. (a) Representative traces of phospholipid scrambling by afTMEM16 with 0 nM (black), 100 nM (green), 250 nM (mustard), 500 nM (blue), 1 μM (pink), 2.5 μM (cyan), 5 μM (brown) and 0.5 mM Ca2+(red). For clarity, only values ofF/Fmaxbetween 0.1 and 0.5 are shown. (b) Ca2+-dependence ofAFast(black circles) andASlow(red squares). Solid lines represent fits to a Hill equation withKmApp(Fast)=0.44±0.13 μM,n(Fast)=1.2±0.4 andKmApp(Slow)=0.44±0.07 μM,n(Slow)=1.5±0.3. Wild-type (WT) afTMEM16: solid symbols and lines; D511A/E514A mutant: empty symbols and dashed lines. Each data point represents the average of 8–12 independent experiments. (c) Average Cl−trapped in liposomes with WT afTMEM16 or the D511A/E514A mutant as a function of Ca2+. Each data point represents the average of 5–17 independent experiments. (d–f) Divalent selectivity of phospholipid scrambling (d,e) and ion channel activity of afTMEM16 (f). In all cases, the colour coding is as follows: 0 mM Ca2+(black), 0.3 mM Ca2+(red), Mn2+(green), Sr2+(blue), Ba2+(pink), Cd2+(cyan) or Mg2+(brown). (d) Representative traces of fluorescence decay upon addition of dithionite. (e) AverageF*=F(t=3τ0)/FMaxin the presence of divalent cations. Each data point represents the average of five to ten independent experiments. (f) Average % of trapped Cl−in afTMEM16 in the presence of divalent cations. Each data point represents the average of 7–12 independent experiments. (g,h) Representative traces of phospholipid scrambling (g) or Cl−efflux (h) mediated by the D511A/E514A mutant with 0.5 (red) or 0 (black) mM Ca2+. Average values ofAFastandASlowfor the D511A/E514A mutant in 0 and 0.5 mM Ca2+are shown inb. ^Addition of Valinomycin. Scale bar, 20 s. For all data points, the error bars are the s.e.m. The errors on the fit parameters are the uncertainties of the fits. Figure 3: A shared Ca2+ binding site regulates channel gating and phospholipid scrambling by afTMEM16. ( a ) Representative traces of phospholipid scrambling by afTMEM16 with 0 nM (black), 100 nM (green), 250 nM (mustard), 500 nM (blue), 1 μM (pink), 2.5 μM (cyan), 5 μM (brown) and 0.5 mM Ca 2+ (red). For clarity, only values of F / F max between 0.1 and 0.5 are shown. ( b ) Ca 2+ -dependence of A Fast (black circles) and A Slow (red squares). Solid lines represent fits to a Hill equation with K m App (Fast)=0.44±0.13 μM, n (Fast)=1.2±0.4 and K m App (Slow)=0.44±0.07 μM, n (Slow)=1.5±0.3. Wild-type (WT) afTMEM16: solid symbols and lines; D511A/E514A mutant: empty symbols and dashed lines. Each data point represents the average of 8–12 independent experiments. ( c ) Average Cl − trapped in liposomes with WT afTMEM16 or the D511A/E514A mutant as a function of Ca 2+ . Each data point represents the average of 5–17 independent experiments. ( d – f ) Divalent selectivity of phospholipid scrambling ( d , e ) and ion channel activity of afTMEM16 ( f ). In all cases, the colour coding is as follows: 0 mM Ca 2+ (black), 0.3 mM Ca 2+ (red), Mn 2+ (green), Sr 2+ (blue), Ba 2+ (pink), Cd 2+ (cyan) or Mg 2+ (brown). ( d ) Representative traces of fluorescence decay upon addition of dithionite. ( e ) Average F *= F ( t =3 τ 0 )/ F Max in the presence of divalent cations. Each data point represents the average of five to ten independent experiments. ( f ) Average % of trapped Cl − in afTMEM16 in the presence of divalent cations. Each data point represents the average of 7–12 independent experiments. ( g , h ) Representative traces of phospholipid scrambling ( g ) or Cl − efflux ( h ) mediated by the D511A/E514A mutant with 0.5 (red) or 0 (black) mM Ca 2+ . Average values of A Fast and A Slow for the D511A/E514A mutant in 0 and 0.5 mM Ca 2+ are shown in b . ^Addition of Valinomycin. Scale bar, 20 s. For all data points, the error bars are the s.e.m. The errors on the fit parameters are the uncertainties of the fits. Full size image We then purified the afTMEM16 mutant D511A/E514A in which we charge-neutralized a conserved di-acidic motif ( Supplementary Fig. S1 ) that was shown to be critical for the Ca 2+ sensitivity of TMEM16A and TMEM16F [8] , [35] . This mutant mediates Ca 2+ -independent scrambling ( Fig. 3g ), at lower rates than the wild-type protein in 0 mM Ca 2+ . Similarly, liposomes reconstituted with the D511A/E514A mutant retained ~80% of their Cl − content in 0.5 or 0 mM Ca 2+ , indicating that this channel is not activated by Ca 2+ ( Fig. 3c,h ). Therefore, a single, evolutionarily conserved, Ca 2+ -binding site appears to regulate ion and lipid transport. afTMEM16 forms separate pathways for ions and lipids To determine whether afTMEM16 forms independent pathways for ions and lipids, or whether the two substrates permeate through a single transmembrane pore, we exploited our observation that the channel activity of afTMEM16 is modulated by its lipid environment. We noticed that in membranes formed from a 3:1 mixture of POPE (1-palmitoyl-2-oleoyl PE) and 1-palmitoyl-2-oleoyl phosphatidylglycerol (POPG; PE/PG), the afTMEM16 channel is poorly active: out of 263 attempts, we recorded channel activity only seven times ( Supplementary Table S2 ); these recordings were also brief, with only three of them lasting longer than 3 min ( Supplementary Table S2 ). In contrast, the flux assays show that the afTMEM16 channel is fully active in liposomes formed from a 3:1 mixture of E. coli polar lipids and egg PC (Coli/PC) ( Fig. 2b,c ). We tested whether this different activity was due to the diverse lipid composition, by measuring fluxes mediated by afTMEM16 in liposomes formed from the PE/PG mixture. We found that these proteoliposomes retain most of their Cl − content, regardless of the presence of saturating Ca 2+ ( Fig. 4a ), 86±4% ( n= 6) and 69±8% ( n= 6), respectively, in the absence and presence of Ca 2+ . Thus, in PE/PG membranes the channel activity of afTMEM16 is severely inhibited. When we attempted to record afTMEM16 channels in planar lipid bilayers formed from Coli/PC lipids, we found that they are unstable, lasting <5 min on average ( Supplementary Table S2 ) and are thus unsuitable for electrophysiological recordings. Despite this, we did see channels with properties similar to those seen in PE/PG bilayers (high conductance and poor selectivity) in 2 out of 18 attempts ( Supplementary Table S2 ), suggesting that the channel is more active in these conditions. Further work is necessary to identify a lipid composition suitable for the electrophysiological characterization of afTMEM16. Despite these limitations, our results suggest that the lipid composition of the membrane is a critical regulator of the activity of afTMEM16 as an ion channel. In contrast, the Ca 2+ -dependent scramblase activity of afTMEM16 is nearly unaffected by its lipid environment: the kinetics of fluorescence decay in PE/PG liposomes are only ~2-fold slower than those seen in Coli/PC vesicles ( Fig. 4b ), and this mild reduction is reflected in F *-values that are slightly higher than those seen in Coli/PC vesicles ( Supplementary Fig. S9c ). Thus, the PE/PG membrane scaffold drastically inhibits the channel activity of afTMEM16 but has only a minor effect on its ability to scramble lipids, suggesting that afTMEM16 forms physically separate pathways for ions and lipids ( Fig. 4d ). This conclusion predicts that preventing ion flux, for example, by replacing K + with an impermeant ion, should not affect the rate of lipid transport. This is the case: afTMEM16 mediates Ca 2+ -dependent scrambling in the presence of the impermeant NMDG + ion ( Fig. 4c and Supplementary Fig. S9d ), with kinetics comparable to those observed in K + ( Fig. 1g ). As noted above, vesicles prepared in NMDG-Cl appear to have a larger refractory pool, ~30% ( n= 6), than vesicles prepared in KCl, ~20%, as evinced by the higher value of the steady-state level of fluorescence in these conditions ( Fig. 4c ). 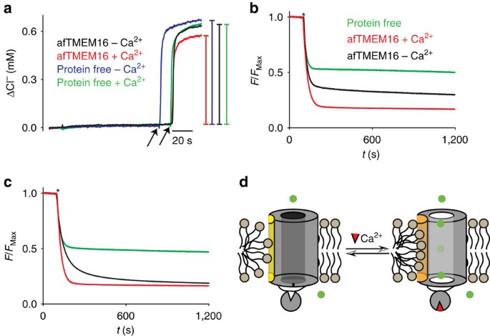Figure 4: Separation of the ion and lipid pathways of afTMEM16. (a,b) Representative traces of Cl−efflux (a) or phospholipid scrambling (b) by afTMEM16 in PE/PG liposomes with 0.5 (red) or 0 (black) mM Ca2+. Traces corresponding to protein-free liposomes in the absence (blue) or presence of Ca2+(green) are also shown. Scale bar, 20 s. Arrows denote addition of detergent to solubilize liposomes. (c) Representative traces of phospholipid scrambling by afTMEM16 in NMDG+with 0.5 (red) or 0 (black) mM Ca2+. (d) Cartoon representation of the structural bases of the dual function of afTMEM16. With no Ca2+, the channel is closed (black) and the lipid pathway (yellow) is partly occluded. Ca2+(red) binding to a single site opens the channel (white) and lipid pathway (mustard). Figure 4: Separation of the ion and lipid pathways of afTMEM16. ( a , b ) Representative traces of Cl − efflux ( a ) or phospholipid scrambling ( b ) by afTMEM16 in PE/PG liposomes with 0.5 (red) or 0 (black) mM Ca 2+ . Traces corresponding to protein-free liposomes in the absence (blue) or presence of Ca 2+ (green) are also shown. Scale bar, 20 s. Arrows denote addition of detergent to solubilize liposomes. ( c ) Representative traces of phospholipid scrambling by afTMEM16 in NMDG + with 0.5 (red) or 0 (black) mM Ca 2+ . ( d ) Cartoon representation of the structural bases of the dual function of afTMEM16. With no Ca 2+ , the channel is closed (black) and the lipid pathway (yellow) is partly occluded. Ca 2+ (red) binding to a single site opens the channel (white) and lipid pathway (mustard). Full size image We identified a novel homologue of the TMEM16 family of channels that is a dual-function protein: it is a Ca 2+ -gated ion channel and a Ca 2+ -dependent lipid scramblase. Not all TMEM16 family members share this dual functionality, indicating that the family is evolutionarily divided between ion channels and dual-function channel/scramblases. Our results suggest that afTMEM16 has a remarkable structural architecture in which a single Ca 2+ -binding site regulates two distinct pathways ( Fig. 4d ). All TMEM16 family members have the same number of transmembrane domains ( Supplementary Fig. S1 ), regardless of whether they are just ion channels, only scramblases or have both functions. This rules out the simple idea that a ‘scramblase module’ was appended to a channel, or vice versa. In contrast, the functional divergence of the TMEM16 family appears to be built on a single structural framework and that subtle alterations, accumulated through evolution, resulted in the formation of a lipid-specific transmembrane pathway in addition to the conserved ion pore. Indeed, the transmembrane (TM), domains that presumably line the ion-channel pore [6] , [8] , [35] are well conserved in the TMEM16 family ( Supplementary Fig. S1 and Supplementary Table S1 ). In contrast, the poor conservation of the other transmembrane regions ( Supplementary Fig. S1 ) might offer a hint as to the localization of the lipid pathway. We propose that the separation of the pathways underlies the evolutionary divergence in the TMEM16 family: mutations in one will have little or no effect on the other, allowing the two pathways to evolve separately. This hypothesis is supported by a recent report that shows that heterologous overexpression of several other TMEM16 homologues is associated with Ca 2+ -dependent PL scramblase activities but not with ion channel function [13] , suggesting that this functional diversity might be a general characteristic of the TMEM16 family. It is remarkable that a single, evolutionarily conserved Ca 2+ -binding site controls opening of the TMEM16 ion and lipid pathways, suggesting that the structural elements gating the two pathways are shared. The hypothesis that the pathways, although spatially separate, share common gating elements is supported by the observation that in PE/PG membranes the ion channel activity of afTMEM16 is abolished while its ability to scramble lipids suffers only a minor reduction in rate. Our finding that afTMEM16 is both a Ca 2+ -gated ion channel and a Ca 2+ -dependent scramblase suggests that TMEM16F might also be a dual-function channel/scramblase, rather than being just a scramblase [13] , or an ion channel that regulates a scramblase [8] . This implies that other, Ca 2+ -independent, scramblases exist. Indeed, platelets from a Scott syndrome patient retain a TMEM16F-independent pathway for PS exposure in normal and apoptotic condition [10] . The molecular identification of these scramblases remains an objective for future work. Cloning and purification of afTMEM16 We renamed the A. fumigatus AFUA_4G02970 gene ( Aqy1 , PubMed gene ID: 3504033) to afTMEM16 for consistency with other TMEM16 proteins. The afTMEM16 and IST2 genes were codon-optimized for overexpression in yeast (GenScript, USA), cloned into the S. cerevisiae Uracil-selectable yEGFP-fusion vector pDDGFP2 (ref. 40 ) and expressed as C-terminally yEGFP-His8-tagged fusion proteins under control of the GAL1 promoter. A Tobacco Etch Virus protease site between afTMEM16 and the yEGFP-His8 tag allows for tag removal. The afTMEM16 D511A/E514A mutant was generated using the Quickchange method (Agilent) and was fully sequenced. The vector was transformed into S. cerevisiae FYG217-competent cells [40] carrying a URA3 deletion for positive selection. Cells were grown in yeast synthetic drop-out medium supplemented with Uracil (CSM-URA; MP Biomedicals). Expression was induced with 2% (w/v) galactose at 30 °C and monitored by green fluorescent protein fluorescence detection and western blotting, with anti-green fluorescent protein and anti-His antibodies (Santa Cruz Biotechnology). Cells were collected after 22 h and lysed in an EmulsiFlex-C5 homogenizer at 25,000 psi in buffer P (150 mM KCl, 10% (w/v) glycerol, 50 mM Tris-HCl, pH 8) supplemented with 1 mM EDTA, 5 μg ml −1 leupeptin, 2 μg ml −1 pepstatin, 100 μM phenylmethane sulphonylfluoride and protease inhibitor cocktail tablets (Roche). Extraction was carried out by adding digitonin (EMD Biosciences) for afTMEM16 and Foscholine 12 (Affymetrix) for Ist2p, to 1% (w/v) for 1–2 h at 4 °C with gentle mixing. After centrifugation at 40,000 g for 45 min, 1 mM MgCl 2 and 10 mM Imidazole were added, the supernatant was loaded on a Ni-NTA agarose resin (Qiagen), washed with buffer P+30 mM Imidazole and 0.12% (w/v) digitonin (0.1% w/v Foscholine 12 for Ist2p), and eluted with buffer P+300 mM Imidazole and 0.12% (w/v) digitonin (0.1% w/v Foscholine 12 for Ist2p). After overnight treatment with Tobacco Etch Virus protease to remove the His tag, the protein was run on a Superdex 200 column (GE Healthcare) with buffer P containing 0.12% (w/v) digitonin (0.1% w/v Foscholine 12 for Ist2p), and the peak fraction containing afTMEM16 was collected. Liposome preparation Liposomes were formed from a 3:1 (mol/mol) mixture of Coli/PC, or a 3:1 mixture of PE/PG (Avanti Polar Lipids). Lipids were dissolved in buffer L (300 mM KCl, 20 mM HEPES, 0.5 mM Ca(NO 3 ) 2 or 1 mM EGTA, pH 7.4; unless otherwise stated) and 35 mM 3-[(3-cholamidopropyl)dimethylammonio]-1-propanesulfonate (CHAPS). Purified protein was added to the detergent/lipid suspension to the desired protein density (5 μg protein per mg lipid, unless otherwise stated). Detergent was removed by dialysis (4 changes at 1,000 × volume of buffer L over 36 h at 4°C) or using Bio-beads (4 changes of 200 mg Bio-beads SM-2 adsorbent (Bio-Rad) per ml of liposomes pre-equilibrated with buffer L and incubated at 4 °C with gentle rotation for 48 h). Liposomes were collected, flash frozen in liquid nitrogen and stored at −80°C. Both methods gave comparable results in both Cl − flux and lipid scrambling assays. Preparation of the Ca 2+ solutions The free [Ca 2+ ] present in our standard solution (300 mM KCl, 20 mM HEPES, pH 7.4) was measured with a Ca-sensitive electrode (Orion Research, Inc.), and was found to be 55±5 μM. The amounts of Ca 2+ and EGTA to generate the desired free Ca 2+ concentrations were calculated using the program Ca-EGTA Calculator v1.3, from the website ( http://www.stanford.edu/~cpatton/CaEGTA-TS.htm ) and the values were verified (for [Ca 2+ ] free >1 μM) using the Ca-sensitive electrode. For solutions containing less than 1 μM [Ca 2+ ] free the predicted value was used. Our 0 mM Ca 2+ solution was obtained by adding 1 mM EGTA to the standard solution for a predicted [Ca 2+ ] free of ~8 nM. Flux assay Liposomes were extruded through a 400-nm membrane filter and centrifuged through a Sephadex G-50 column (Sigma-Aldrich) pre-equilibrated in the desired external buffer (1 mM KCl, 300 mM Na-glutamate, 20 mM HEPES, 0.5 mM Ca(NO 3 ) 2 , pH 7.4). One hundred microlitres of liposomes were diluted in 2 ml of buffer and the Cl − time course was monitored with an AgCl electrode. After baseline stabilization, 1 μl of the K + ionophore Valinomycin (2 mg ml −1 ) was added to test whether Cl − efflux could be initiated. The experiment was terminated after 90 s by addition of 40 μl of 1.5 M n-octyl-β- D -glucopyranoside (Affymetrix) to dissolve liposomes and determine the total Cl − content of the liposomes, ΔCl − . For each experiment, ΔCl − was normalized to the average Cl − content of 3+ experiments with protein-free liposomes in the presence of 0.5 mM Ca 2+ prepared from the same batch of lipids. Planar lipid bilayer recordings Horizontal planar lipid bilayers [41] were formed from decane solutions of PE/PG or Coli/PC lipids at 10 mg ml −1 . The cis -chamber contained 300 mM KCl, 20 mM HEPES and 0.5 mM Ca(NO 3 ) 2 , pH 7.4, and the trans -chamber contained 30 mM KCl, 20 mM HEPES and 0.5 mM Ca(NO 3 ) 2 , pH 7.4. Proteoliposomes (in the presence of 0.5 mM Ca(NO 3 ) 2 ) were sonicated for 5 s, and 1 μl was added to the cis- chamber. Bilayer formation was monitored by measuring the capacity using a triangular wave; acceptable capacities were 70–110 pF. After addition of 1 μl of liposomes, 1 μl of 3 M KCl was added to promote fusion [41] . Successful incorporation of channels was monitored by holding at −100 or +100 mV. Bilayer capacity was periodically checked. The minimum wait time for channel incorporation was 10 min. Bilayers formed from the Coli/PC mix proved to be unstable and, on average, lasted<5 min from formation. Currents were recorded using the GePulse software (by M. Pusch, Istituto di Biofisica, Genova, Italy) with a Whole Cell/Patch Clamp Amplifier PC-505B (Warner Instruments) sampled at 1 ms and filtered at 1 kHz. Lipid scrambling Liposomes were prepared as described above, except that trace amounts of NBD-PLs (0.5% of total lipid weight) were included. Scrambling activity was assayed as described previously [24] . Briefly, liposomes were loaded with 300 mM KCl, 20 mM HEPES and 0.5 mM Ca(NO 3 ) 2 , pH 7.4. Ca 2+ concentrations were adjusted as described. Liposomes were extruded through a 400-nm membrane filter, and 20 μl were diluted to 2 ml in 300 mM KCl, 50 mM HEPES, X mM Ca(NO 3 ) 2 , pH 7.4 in a stirred cuvette at 23 o C and the fluorescence intensity (excitation 470 nm, emission 530 nm) was recorded in a PTI spectrofluorimeter. Forty microlitres of sodium dithionite (40 mM final concentration) or fatty-acid-free BSA (1.5 mg ml −1 final concentration) were added to the cuvette to start the reaction. Data was collected using FelixGX 4.1.0 at a sampling rate of 1 or 3 Hz. Analysis of the time course of fluorescence decay The general form of the model describing the dithionite-induced fluorescence decay of proteoliposomes containing a single scramblase is a three-state scheme where L * in/out denote the fluorescent form of the lipid in the inner (outer) leaflet and L is the dithionite-reduced non-fluorescent form, κ ±1 are the forward and backward rates of scrambling and κ 2 is the rate of dithionite reduction. As this is a three-state system, the time evolution of L * in ( t ), L * out (t) and L ( t ) is described by a double exponential [42] . The time course of the normalized fluorescence is which was fitted to where A 0 is an offset needed to account for the fraction of refractory liposomes, A Fast(Slow) is the relative weight of the fast (slow) component of the decay and τ Fast(Slow) is its relative time constant. It is important to note that A Fast(Slow) and τ Fast(Slow) are complex functions of the rates of scrambling and of dithionite reduction, and therefore do not represent distinct physical processes. For [Ca 2+ ]<1 μM, the trace is well fit with a double exponential. For [Ca 2+ ]>5 μM, the process is well described by a single exponential, as A Slow becomes ~0. Poisson analysis Assuming that the reconstitution process randomly inserts proteins into liposomes, the fraction of liposomes containing 0 copies of a protein, f 0 , is given by Poisson statistics where N P and N L are the number of proteins and liposomes in the sample, p is the protein density, , γ is the number of liposomes per mass of lipid, M P is the mass of the functional protein complex, ϕ is the fraction of active proteins and N A is Avogadro’s number [26] . In our analysis, we assumed that ϕ ~1 and used the experimentally derived values of γ reported in the literature [26] . To compare the f 0 -values obtained from assays with different dynamical ranges (fluxes, dithionite and scrambling), the data were normalized as follows: where y 0 is the signal measured with protein-free liposomes, y max is the signal at 5 μg protein per mg lipid and y is the signal measured at each protein concentration. Sequence alignments Amino acid sequences of TMEM16A, B, E, F and afTMEM16 were aligned with the M-Coffee program [43] , which combines several multiple alignment programs in single output. E -values for TM1, 2, 5 and 7a/b from afTMEM16 with the corresponding domains from TMEM16A, B, E, F and Ist2p, respectively, were obtained using DELTA-Blast ( http://blast.ncbi.nlm.nih.gov ). The boundaries of the individual TM domains were chosen as described in Supplementary Fig. S2 . For the other four TM domains (TM3, 4, 6 and 8), no significant alignment scores were obtained because of their short length and low degree of homology. Data analysis and statistics Data were analysed using the Ana software (by M. Pusch), Microsoft excel and SigmaPlot 10.0. The experiments were repeated 3–20 times, exact numbers are reported in the text or in the figure legends. Data points are reported as mean±s.e.m. The error reported for parameters derived from fits is the uncertainty of the fit rather than the s.e.m. How to cite this article: Malvezzi, M. et al . Ca 2+ -dependent phospholipid scrambling by a reconstituted TMEM16 ion channel. Nat. Commun. 4:2367 doi: 10.1038/ncomms3367 (2013).